Deoxygenation alters bacterial diversity and community composition in the ocean’s largest oxygen minimum zone Oceanic oxygen minimum zones (OMZs) have a central role in biogeochemical cycles and are expanding as a consequence of climate change, yet how deoxygenation will affect the microbial communities that control these cycles is unclear. Here we sample across dissolved oxygen gradients in the oceans’ largest OMZ and show that bacterial richness displays a unimodal pattern with decreasing dissolved oxygen, reaching maximum values on the edge of the OMZ and decreasing within it. Rare groups on the OMZ margin are abundant at lower dissolved oxygen concentrations, including sulphur-cycling Chromatiales , for which 16S rRNA was amplified from extracted RNA. Microbial species distribution models accurately replicate community patterns based on multivariate environmental data, demonstrate likely changes in distributions and diversity in the eastern tropical North Pacific Ocean, and highlight the sensitivity of key bacterial groups to deoxygenation. Through these mechanisms, OMZ expansion may alter microbial composition, competition, diversity and function, all of which have implications for biogeochemical cycling in OMZs. Throughout the global ocean, biological material that sinks out of the euphotic zone is remineralized and respired by microbial communities at depth. Microbial respiration concurrently consumes dissolved oxygen (DO), and can deplete DO below 20 μmol kg −1 in areas of high primary production and sluggish ventilation of subsurface waters [1] . These low DO concentrations [2] delineate oxygen minimum zones (OMZs) found in the Arabian Sea, the Eastern tropical South Pacific Ocean (ETSP), and the Eastern tropical North Pacific Ocean (ETNP). Large aerobic organisms are mostly absent from OMZs [3] , but anaerobic microbial processes are active, and OMZs consequently have an important role in global biogeochemical cycles [4] , [5] , [6] , [7] . However, both the volume of OMZs and the biogeochemical processes occurring within them are highly sensitive to anthropogenic climate change: OMZs are warming, expanding and being further depleted of oxygen [1] , [3] , [8] , while model results indicate that anaerobic nitrogen (N) loss from the ETNP has varied fourfold in response to twofold changes in suboxic water volume during the past 50 years [7] . These findings suggest that biogeochemical and ecological responses to ocean warming and deoxygenation are rapid and nonlinear, yet no long time series and few experimental studies exist [9] , [10] . The major OMZs are also characterized by only a handful of studies examining microbial diversity at 3–8 depths at 1–3 stations [10] , [11] , [12] , [13] , [14] . How deoxygenation will affect OMZ microbial communities and processes is therefore poorly understood. Biogeochemically, OMZ expansion may increase global N loss [4] , [7] , but our understanding of N and sulphur (S) cycling in OMZs is still evolving [4] , [5] , [6] . At the community level, microbial diversity in the ETSP was originally thought to increase as oxygen decreased with depth [12] , but more recent data display an opposing pattern [10] . Alternatively, microbial diversity might peak at mid-depths—where biogeochemical cycling of carbon (C), N and S is rapid and dynamic—and previous coarse-grained sampling may have missed this peak [10] , [15] . This is an important distinction, because the upper ocean will remain well-lit, warm, mixed and oxygenated as the climate changes: if microbial diversity and composition display monotonic successional patterns along depth gradients, these patterns may simply steepen as OMZs shoal upwards. In contrast, unimodal patterns indicate that diversity is not a linear function of depth, temperature, light, oxygen or nutrients. This may reflect individual responses among operational taxonomic units (OTUs) and functional groups to these or other variables, and/or non-linear responses to multiple variables. For example, phototrophic organisms may track light gradients, heterotrophic groups may track organic C availability, N-cyclers may track N availability, and aerobes and anaerobes will be strongly affected by variations in DO. Their collective variations define overall diversity and composition. Here we hypothesize that microbial diversity is greatest in the ETNP either at the base of euphotic zone, where sinking organic material provides chemical energy to fuel microbial metabolism [10] , or on the edge of OMZs, where availability of oxidants and reductants may generate functional and taxonomic diversity [12] . In either case, where OMZs reach the base of the euphotic zone, low DO might reduce diversity among aerobes due to varying oxygen tolerances [10] . OMZ shoaling may also alter competition for resources—especially through availability of light within the OMZ, which could favour photoauto- and photohetero-trophs in the competition for nutrients and substrates [16] . Within the OMZ, further decreases in DO may favour particular groups and particular forms of metabolism. These changes are not mutually exclusive, and could act together to alter microbial distributions, diversity and composition. As these changes in communities can have demonstrable effects on biogeochemical cycling of C (refs 17 , 18 , 19 ) and N (ref. 20 ), we investigate bacterial community ecology in the OMZ of the Gulf of California (GOC; the body of water defined by the Baja California peninsula and mainland Mexico) and ETNP using pyrosequencing of 16S rRNA genes. Our findings indicate that bacterial richness peaks on the edge of the OMZ, and along with community composition, is a strong function of DO. Our quantitative analysis of these data supports the idea that OMZ expansion and deoxygenation can alter bacterial distributions, diversity and composition through the mechanisms above. Trends in DO We sampled the Carmen Basin of the GOC (station 1; Fig. 1 ), the mouth of the GOC (station 2), and in the ETNP OMZ (station 3), where DO concentrations declined rapidly to 20 μmol kg −1 by 111 m. Three additional stations extended north from the tip of Baja California (stations 4–6). Measured DO concentrations were lower at nearly every depth at stations 2–6 compared with data from the 2005 World Ocean Atlas (WOA; Fig. 1 ). DO appeared to increase only at station 1, and WOA data indicate that seasonal DO changes are not prevalent in the ETNP [2] . Following Stramma et al . [3] , [8] , we integrated DO over 300–700 m depth and compared our cruise data with historical data from the California Cooperative Oceanic Fisheries Investigations (CalCOFI); we calculated that integrated DO loss ranged from 87±61 to 302±103 mmol m −2 per year, slightly higher than reported rates of OMZ deoxygenation of 37–136 mmol m −2 per year (ref. 8 ). Comparing each station with the station immediately north—where the OMZ is less developed—OMZ DO concentrations were 0.1±0.2 to 23.9±1.4 μmol kg −1 lower, and DO was higher only at 400 m at station 5 compared with station 6 ( Fig. 1 ). These values are similar to differences in DO between cruise data and WOA data for individual stations, which ranged from a 11.9±1.6-μmol kg −1 increase to a 20.2±1.3-μmol kg −1 decrease ( Fig. 1 and also for stations 1 and 6). Based on these findings, the spatial differences in DO among stations are comparable to the deoxygenation rates observed at each station. 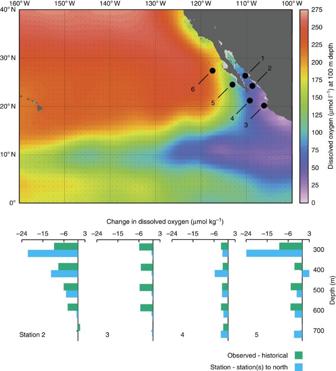Figure 1: Oxygen gradients in the GOC and ETNP. Station locations (numbered black circles) are plotted on DO concentrations (in μmol l−1) at 100 m depth from the World Ocean Atlas. Bottom panels show differences between measured DO concentrations (in μmol kg−1) and historical DO concentrations (green bars), and differences in DO between stations (blue bars), for the 300–700 m depth range. For inter-station comparisons, station 2 is compared with station 1, station 4 with station 5 and station 5 with station 6. Station 3 is compared with both station 2 and station 4, but differences with historical data were much greater than the differences among stations 2–4, hence blue bars are barely visible. Figure 1: Oxygen gradients in the GOC and ETNP. Station locations (numbered black circles) are plotted on DO concentrations (in μmol l −1 ) at 100 m depth from the World Ocean Atlas. Bottom panels show differences between measured DO concentrations (in μmol kg −1 ) and historical DO concentrations (green bars), and differences in DO between stations (blue bars), for the 300–700 m depth range. For inter-station comparisons, station 2 is compared with station 1, station 4 with station 5 and station 5 with station 6. Station 3 is compared with both station 2 and station 4, but differences with historical data were much greater than the differences among stations 2–4, hence blue bars are barely visible. Full size image Although no approach can completely mimic large-scale global changes such as ocean deoxygenation, use of natural gradients to ‘substitute space for time’ is a robust approach for modelling ecological responses to environmental change [21] ; ocean deoxygenation research has examined the distribution of organisms along oxygen gradients in present OMZs, and related these data to historical deoxygenation [3] . Our approach is analogous, and our OMZ transect captures variation in DO with limited variation in other respects. In particular, primary production rates were similar at the time of our sampling (27–34 mmol m −2 d −1 at stations 2–4 and 6, 47 mmol m −2 d −1 at station 5, and 67 mmol m −2 d −1 at station 1; ref. 22 ), and long-term satellite-based chlorophyll measurements showed few differences ( Supplementary Discussion ). Temperature did decline with increasing latitude—reaching ~30 °C at the surface at station 3 but 21 °C at station 6—as well as with increasing depth ( Supplementary Fig. S1 ). As deoxygenation scales with temperature change [1] , and DO and temperature decrease in parallel in the ocean ( Supplementary Fig. S2 ; Supplementary Discussion ), we analysed relationships between both DO and temperature and bacterial diversity. Patterns in diversity At most stations, richness and evenness were low in the euphotic zone ( Fig. 2 and Supplementary Fig. S3 ), and the cyanobacteria Prochlorococcus and Synechococcus frequently dominated these libraries, constituting up to 74% of 16S rRNA sequences (station 1, 25 m library; Fig. 3 ). Richness reached higher values at the base of the euphotic zone, and then decreased with depth between the euphotic zone and OMZ. For example, the second highest ACE values were located within 0–14 m of the 1% light level at stations 2, 3, 4 and 6 (55–66 m; Fig. 2 ), but relatively low values were subsequently found at 100 m at stations 3, 4 and 6. At all stations, ACE-estimated richness reached maximum values at the top of the OMZ ( Fig. 2 and Supplementary Fig. S3 ). This was a consistent feature in the GOC and ETNP, as richness peaked at different depths at different stations, and consequently tracked changes in DO profiles between stations. Moving across the transect, peak ACE-estimated richness occurred at 400 m at station 1, 100 m at station 2, 120 m at station 3, 140 m at station 4, and 200 m at stations 5 and 6 ( Fig. 2 ). Observed richness exhibited similar patterns ( Supplementary Fig. S3 ). Estimated richness peaked at oxygen concentrations of 9.1–15.3 μmol kg −1 at stations 1, 4, 5 and 6, and at slightly lower DO values at stations 2 (8.4 μmol kg −1 ) and 3 (6.4 μmol kg −1 ). However, along the steep oxygen gradients present at stations 2 and 3, DO changes by >14 μmol kg −1 within 10 m depth ( Fig. 2b,c ), and a small change in sampling depth would yield DO values more similar to the other stations. 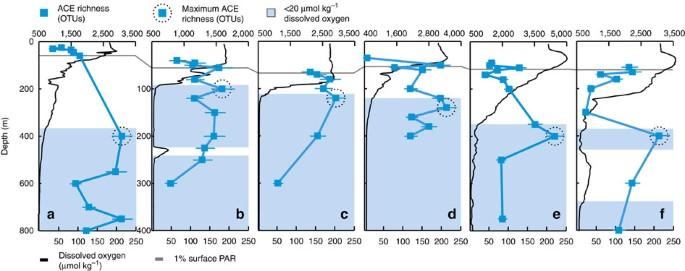Figure 2: Depth profiles of ACE-estimated richness. Data are from normalized libraries from station 1 (a), 2 (b), 3 (c), 4 (d), 5 (e) and 6 (f). ACE values (blue squares) are shown on the upper horizontal axis (note the difference among scales) and error bars denote 95% confidence intervals. Samples containing maximum community richness are circled (dotted circle). Vertical axes indicate depth in the water column; data from station 1 extend to 800 m, whereas stations 2–6 are plotted on the same axis to 400 m depth. DO profiles are displayed by the solid black lines, with values (μmol kg−1) shown along the lower axis of plotsa–f. The OMZ (<20 μmol kg−1DO) is shown by blue shading. The depth of the euphotic zone is denoted by the level of 1% surface photosynthetically active radiation (PAR) and the grey line in panelsa–f. Figure 2: Depth profiles of ACE-estimated richness. Data are from normalized libraries from station 1 ( a ), 2 ( b ), 3 ( c ), 4 ( d ), 5 ( e ) and 6 ( f ). ACE values (blue squares) are shown on the upper horizontal axis (note the difference among scales) and error bars denote 95% confidence intervals. Samples containing maximum community richness are circled (dotted circle). Vertical axes indicate depth in the water column; data from station 1 extend to 800 m, whereas stations 2–6 are plotted on the same axis to 400 m depth. DO profiles are displayed by the solid black lines, with values (μmol kg −1 ) shown along the lower axis of plots a – f . The OMZ (<20 μmol kg −1 DO) is shown by blue shading. The depth of the euphotic zone is denoted by the level of 1% surface photosynthetically active radiation (PAR) and the grey line in panels a – f . 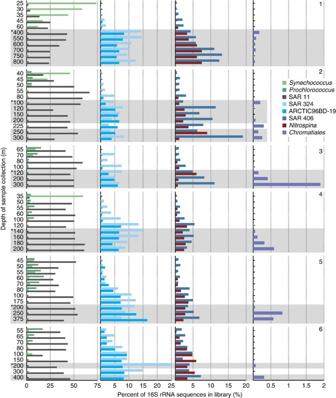Figure 3: Distribution of microbial groups in pyrosequencing libraries. Depth of sample collection is shown along the vertical axis (not to scale), with stations proceeding in order (1–6) from top to bottom. Different colours denote different clades or groups, with each group’s percentage of the total sequences in each library indicated by the bottom axes. Asterisks denote libraries of maximum estimated richness, and grey shading denotes samples collected within the OMZ. Full size image Figure 3: Distribution of microbial groups in pyrosequencing libraries. Depth of sample collection is shown along the vertical axis (not to scale), with stations proceeding in order (1–6) from top to bottom. Different colours denote different clades or groups, with each group’s percentage of the total sequences in each library indicated by the bottom axes. Asterisks denote libraries of maximum estimated richness, and grey shading denotes samples collected within the OMZ. Full size image From peak values at the top of the OMZ, richness declined with increasing depth and decreasing DO. This pattern was most distinct at stations 2 and 3, where the lowest overall richness was found at 300 m in the OMZ, rather than within the euphotic zone ( Fig. 2b,c ). In comparing richness data from all stations with DO concentrations, observed and estimated richness were inversely related with DO outside the OMZ, but were positively related with DO concentrations below 20 μmol kg −1 ( Fig. 4a,b ). The maximal information coefficient (MIC) was recently developed to assess these and other nonlinear relationships [23] , and indicated that variation in four metrics of diversity corresponded to variations in DO and temperature ( Table 1 ). Relationships between DO and diversity were less linear than those based on temperature, with ACE-estimated richness and the Gini coefficient providing the greatest contrast: ACE exhibited a high MIC and was least linear with DO, whereas the Gini coefficient displayed a high MIC and the greatest linearity with temperature. The Gini coefficient is a measure of inequality for which higher values represent a less equal distribution of species abundances [20] ; compared with richness, community evenness decreased more moderately in the OMZ ( Fig. 4c , Supplementary Fig. S3 ). 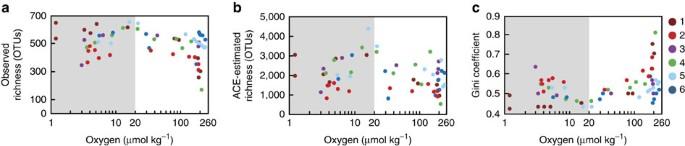Figure 4: Bacterial diversity versus DO. Observed richness (a), ACE-estimated richness (b) and the Gini coefficient (c) are shown in relation to DO (plotted on logarithmic scale). Colours denote data from different stations (see legend), and DO concentrations <20 μmol kg−1are indicated by grey shading. Data are from sequence libraries normalized to 1,298 sequences and OTUs defined by 97% sequence identity. Figure 4: Bacterial diversity versus DO. Observed richness ( a ), ACE-estimated richness ( b ) and the Gini coefficient ( c ) are shown in relation to DO (plotted on logarithmic scale). Colours denote data from different stations (see legend), and DO concentrations <20 μmol kg −1 are indicated by grey shading. Data are from sequence libraries normalized to 1,298 sequences and OTUs defined by 97% sequence identity. Full size image Table 1 Statistics for relationships between DO, temperature and microbial diversity. Full size table We consequently used a variety of statistical approaches to examine the effects of DO and temperature on richness. These analyses demonstrate that DO and temperature have joint, nonlinear effects on richness, with temperature having a greater role in the upper water column, and DO in the lower water column, particularly at low concentrations ( Supplementary Discussion , Table 1 , and Supplementary Table S1 ). For all of these approaches, results from libraries containing 3,000 sequences (which exclude two samples from station 6; see Methods) were similar ( Supplementary Table S1 ). Rarefaction analysis of our sequence data [24] indicated that observed and estimated richness values are clearly significantly different from edge to core in the OMZ, with no overlap among 95% confidence intervals; and that our ACE estimates are likely accurate, as the curves plateau and approach an asymptote ( Supplementary Fig. S4 ). From the edge to the core of the OMZ, observed richness declined by 3.7–39.9%, and ACE-estimated richness decreased by up to 61.9% (at station 3; Supplementary Fig. S4 ), representing differences of thousands of estimated OTUs between samples. Libraries containing 3000 sequences yielded slightly better coverage of observed richness (due to larger libraries) and highly similar ACE estimates ( Supplementary Fig. S5 ). Other OTU definitions support these findings ( Supplementary Table S2 ), which are also unaffected by error-inflated diversity estimates (see Methods). Together these data indicate that variations in bacterial diversity track variations in DO and temperature—both with depth and from station to station—and that richness does not decrease or increase monotonically with depth, but instead peaks on the edge of the OMZ. Variation in bacterial community composition Associated with observed changes in richness, redundancy analysis (RDA) demonstrated that changes in community composition were related to changes in DO and temperature (constrained variance=38%, F =17.8, P <0.05; Fig. 5 ). This is driven by variations in the presence, absence and abundance of multiple OTUs, and we found that 256 OTUs were significantly related to temperature or DO based on MIC. Of these, most relationships were nonlinear, with the majority related to both temperature and DO. Several 16S rRNA sequence types were also rare in the upper OMZ and abundant at greater depths. This included OTUs related to S-oxidizing symbionts, anammox bacteria and the S-cycling Chromatiales (purple sulphur bacteria) ( Supplementary Table S3 ). This supports the idea that the rare biosphere acts as a reservoir of low abundance organisms that increase in numbers under favourable conditions [25] . Chromatiales constituted 1.9% of the bacterial community at 300 m depth at our southernmost station, and exceeded 0.5% of the community in low DO samples collected at stations 3, 4 and 5 ( Fig. 3 ). As an increase in Chromatiales 16S rRNA genes with decreasing DO was observed at these stations, we PCR-screened, and detected, Chromatiales 16S rRNA in extracted RNA from within the OMZ at stations 2–5 ( Fig. 6a ). This is potentially indicative of active protein synthesis, and is consistent with recovery of Chlorobi (green sulphur bacteria) transcripts in the ETSP [14] , where cryptic S cycling occurs. 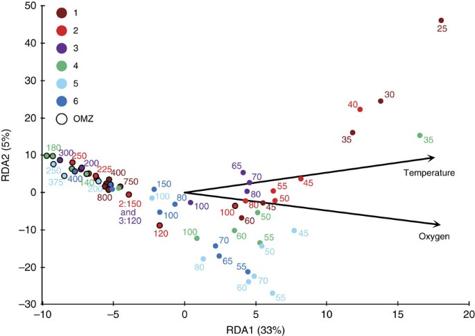Figure 5: Bi-plot of redundancy analysis of bacterial community composition. Colour key denotes different stations, and OMZ datapoints are outlined by a black circle. Depth of sample collection is shown next to most data points; in the OMZ, not all sampling depths are indicated, because some datapoints are obscured by other datapoints and cannot be clearly labelled. Percentage values along axes denote community variation accounted for along the axis; arrows denote biplot scores for the constraining variables, temperature and DO. Figure 5: Bi-plot of redundancy analysis of bacterial community composition. Colour key denotes different stations, and OMZ datapoints are outlined by a black circle. Depth of sample collection is shown next to most data points; in the OMZ, not all sampling depths are indicated, because some datapoints are obscured by other datapoints and cannot be clearly labelled. Percentage values along axes denote community variation accounted for along the axis; arrows denote biplot scores for the constraining variables, temperature and DO. 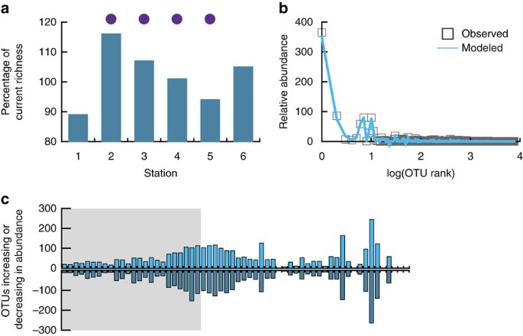Figure 6: MSDM results for the ETNP OMZ. (a) Changes in richness from the MSDM based on historical CalCOFI DO data; stations whereChromatiales16S rRNA was amplified in RNA extracts (see text) are denoted by purple circles. (b) Rank-abundance plot of observed (grey squares) and modelled (blue lines) OTU abundances for 100 m at station 2. For this sample, ther2between observed and modelled abundance is 0.99. (c) Number of OTUs exhibiting increases (light blue) or decreases (dark blue) with simulated deoxygenation of 12 μmol kg−1. Samples are ranked by oxygen concentration along the horizontal axis; DO concentrations <20 μmol kg−1are indicated by grey shading. Full size image Figure 6: MSDM results for the ETNP OMZ. ( a ) Changes in richness from the MSDM based on historical CalCOFI DO data; stations where Chromatiales 16S rRNA was amplified in RNA extracts (see text) are denoted by purple circles. ( b ) Rank-abundance plot of observed (grey squares) and modelled (blue lines) OTU abundances for 100 m at station 2. For this sample, the r 2 between observed and modelled abundance is 0.99. ( c ) Number of OTUs exhibiting increases (light blue) or decreases (dark blue) with simulated deoxygenation of 12 μmol kg −1 . Samples are ranked by oxygen concentration along the horizontal axis; DO concentrations <20 μmol kg −1 are indicated by grey shading. Full size image Putative S-oxidizers [26] from the SAR324 and ARCTIC96BD-19 clades were among the most abundant microbial groups found in the ETNP OMZ, comprising up to 25 and 16.5% of sequence libraries ( Fig. 3 and Supplementary Discussion ). In the Namibian upwelling region, ARCTIC96BD-19, the related SUP05 bacteria, and Sulfurimonas bacteria detoxified sulphide produced in sediments, ‘blooming’ at levels of up to 20% of the picoplankton [5] . ARCTIC96BD-19 reached comparable abundances in the ETNP OMZ (up to 16.5%), but SUP05 and Sulfurimonas were less abundant (<0.4%). Nitrospina 16S rRNA genes formed up to 9% of libraries and correlated with quantitative PCR data ( r 2 =0.79, P <0.05), while nitrite oxidation was detected at the same depths where Nitrospina were numerous [27] . These data indicate that the relative proportions of bacteria within pyrosequencing libraries accurately reflect their proportions within the water column, and, together with amplification of 16S rRNA, are indicative of activity in the ETNP OMZ. Modelling diversity and composition Given these robust patterns and the clear signal of deoxygenation observed at each station, we used multivariate adaptive regression splines (MARS) [28] , [29] to generate microbial ‘species distribution models’ (SDMs) [29] that quantify the abundance of each observed OTU based on multivariate environmental data (Methods). MARS-based SDMs have proven their utility for large organisms [30] , [31] , and here we apply them to microbial communities comprised of thousands of OTUs. This is analogous to the recent work using temperature-based SDMs to model potential phytoplankton diversity [18] , but allows us to calculate the relative abundance of bacterial OTUs based on DO and other environmental variables. As microbial SDMs (MSDMs) model each individual OTU, it is possible to examine both community level changes in richness as the sum changes of multiple OTUs, as well as changes in community structure and composition. These MSDMs allowed us to test several hypotheses related to the overall richness, range and rate of change in abundance of bacterial OTUs in the ETNP. We first tested whether distributions of OTUs and richness patterns would differ based on historical data; we modelled communities based on past DO concentrations in a given water volume, assuming that the modern niche of each OTU reflects its past distribution [29] , [30] . DO concentrations were previously higher at 300–700 m depth at stations 2–6 and past richness is estimated to be 5–70% greater than present richness ( Fig. 6a ). However, decreases in richness over 300–700 m depth can be offset by increases elsewhere, and station 5 provides a clear example of this: past richness was estimated to be 128% of present richness at 300–700 m depth, but 94% of present richness from 20–700 m. Past richness is estimated to be lower at station 1 in the GOC, but historical DO concentrations were lower. These MSDM results highlight the potential for deoxygenation to alter community properties (such as richness) in OMZs by collectively altering abundance patterns of thousands of bacterial OTUs. Much of the modelled change in richness reflects changes in the abundance of rare OTUs, but associated changes in community composition include depth-range expansion or contraction, and changes in the relative abundance of more numerous OTUs. Our MSDM results indicate that 192 OTUs may have expanded their range, whereas 267 OTUs contracted. (We define these as OTUs that, in at least two cases, were previously expected to occur at a given depth but are no longer, as many rare OTUs exhibit this behaviour once). Of the contracting OTUs, those that exhibited sharp changes in range included rare SAR11, Acidobacteria and SAR116 OTUs. A more detailed MSDM based on all data collected by the conductivity–temperature–depth (CTD) sensors—including salinity, photosynthetically active radiation, beam transmission (an index of particle concentrations in the water column), chlorophyll concentrations (based on fluorescence), temperature and DO—had high predictive capacity ( Fig. 6b ; see Methods). We used this to model microbial community composition at 1 m depth resolution at each station in the ETNP. These results show a similar but slightly modified relationship between richness and DO: richness varied from 150–800 OTUs at DO concentrations <15 μmol kg −1 and >100 μmol kg −1 and reached maximum values at ca . 20–60 μmol kg −1 . We subsequently used this MSDM to explore potential effects of future deoxygenation on OMZ bacterial communities by simulating a decrease in DO concentrations of 12 μmol kg −1 . This corresponds to the upper end of average decreases in ocean DO content expected by the year 2100, and lies within many measured declines over the past few decades (reviewed by Keeling et al . [1] ). Other variables were held constant. The MSDM suggests large relative shifts in abundance for many OTUs as a consequence of deoxygenation. In most samples, decreases in the abundance of OTUs were nearly offset by increases in the abundance of other OTUs, and these patterns varied with initial DO concentrations ( Fig. 6 ). Responses were inconsistent where DO is higher in the upper water column, with no expected changes at 55 m at station 2, 45–60 m at station 5, and 55 m at station 6, but large shifts expected at 30 and 45 m at station 1, 35 m at station 4 and 70–80 m at station 6. In contrast, the number of OTUs that increase or decrease in abundance scaled with DO concentrations of 1 to 30 μmol kg −1 . This likely reflects the fact that richness increases with DO across this range, and the fact that the relative changes in low DO samples are smaller (for example, DO can only decrease by a maximum of 5 μmol kg −1 for a 5-μmol kg −1 sample). However, this allows us to calculate the proportional change in richness as a function of deoxygenation. These results indicate that for every 1 μmol kg −1 decrease in DO in the OMZ, 5% of the OTUs will increase or decrease in abundance. We determined which OTUs may be sensitive to dexoygenation by identifying the largest aggregate changes in OTU abundance within the richest samples ( Table 2 ). These data illustrate the complexity of deoxygenation and diversity within individual bacterial groups, as groups such as SAR11, SAR324, SAR406 and the Nitrospina contain some OTUs that may increase with deoxygenation as well as others that may decrease. SAR406 provides a clear example of this, as the SDM indicates that two SAR406 OTUs with higher DO tolerances may decrease in abundance, whereas the largest predicted increase (over threefold) is for a SAR406 OTU that is most abundant at <10 μmol kg −1 DO. Little is known about the SAR406 clade, but the idea that decreasing DO favors SAR406 is supported by Allers et al . [32] , who observed negative correlations between DO and several SAR406 OTUs. A key point is that the shape and slope of these relationships is important in determining which OTUs may increase or decrease in response to deoxygenation. By incorporating this into a quantitative modelling framework, our MSDM results suggest that OTUs within particular bacterial groups may be displaced by other OTUs with differing tolerances or affinities for DO. Table 2 Changes in OTUs with simulated deoxygenation. Full size table Before the advent of molecular techniques, Hutchinson recognized that a fundamental property of the plankton is having its ‘commonest species commoner and all other species rarer,’ and proposed that non-equilibrium conditions generate the ‘paradox of the plankton’ in the open ocean [33] . Our pyrosequencing data from the ETNP support this pattern, and suggest that bacterial communities are most diverse in upper portions of the OMZ. This may be partly driven by non-equilibrium biogeochemical conditions found here: aerobic and anaerobic N cycling processes co-occur at these DO concentrations in OMZ waters of Peru and Namibia [9] , for instance, and ocean deoxygenation may therefore promote diversity in areas where oxygen declines to 20 μmol kg −1 . Put another way, the edge of the OMZ represents a transition zone where aerobes, anaerobes and microaerophiles [34] may all persist and possibly interact. MINE, SDMs and community composition data provide support for this, as many OTUs show either increasing or decreasing trends with DO. In the absence of time series and experiments, our data provide extensive evidence that oxygen is a strong driver of diversity and community composition, and that the range and abundance of individual OTUs is tightly coupled to DO concentrations. However, our data indicate that OMZ expansion will not simply compress vertical gradients in bacterial diversity and community composition: joint dependence on temperature and DO ( Table 1 , Fig. 5 ) demonstrates that multiple environmental factors affect diversity and composition in the ETNP. This is consistent with previous work indicating that temperature has a strong influence on marine microbial diversity [35] , [36] ( Supplementary Discussion ). For instance, Thomas et al . [18] project a 50% decline in phytoplankton diversity in the ETNP associated with future ocean warming. An important distinction between surface and deeper waters is that the signal of ocean warming is detectable but modest at depths below the mixed layer, whereas ocean deoxygenation produces large relative changes in DO within OMZs [1] , [8] . In the ETNP, percentage increases in temperature below 100 m ranged from 0–27%, while DO decreased by 27–77% compared with historical data ( Fig. 1 ). Although connected, warming and deoxygenation are unlikely to proceed at similar paces within and across all OMZs [1] , and MARS-based MSDMs appear particularly effective for examining the effects of interacting changes on microbial communities. Our findings suggest that, as OMZs expand and their upper boundary advances towards the base of the euphotic zone [1] , [8] , OMZ communities will shoal upwards towards euphotic zone communities. This may constrict the most diverse regions of the water column, as well as create OMZ habitat at relatively shallow depths. One interpretation of the contrasting patterns in richness that we observed in the ETNP (unimodal) versus the ETSP (monotonic) is that OMZ waters reach 50 m depth in the ETSP [10] , and that patterns in richness now differ fundamentally from those detected in the ETNP ( Supplementary Table S4 ). Where light reaches the top of the OMZ, a low-light clade of Prochlorococcus is found in the ETSP [37] and Arabian Sea [38] and represents a clear example of differences in OMZ community composition that may be generated by shoaling [16] . Although earlier studies did not generate 16S rRNA sequences to which our data can be compared, we also identified Prochlorococcus OTUs in OMZ samples that were less abundant at shallower depths, as well as a Prochlorococcus OTU that may increase with deoxygenation ( Table 2 ). As OMZs shoal, the relative influences of light and low DO on (photo)heterotrophs are also likely important: light may favour some proteorhodopsin-containing organisms, whereas low DO may favour microaerophiles with high-affinity oxidases [34] . Whether there are bacterial groups capable of exploiting both light and low DO is unknown, but such groups would presumably benefit from OMZ shoaling. In RDA, DO was a strong influence on community composition throughout the water column, and even within the OMZ ( Fig. 5 ). This highlights the fact that although OMZs are defined by DO <20 μmol kg −1 , they are not homogenous: Ulloa et al . [39] recently distinguished AMZs (anoxic marine zones) from OMZs, where AMZs are characterized by nitrite accumulation and active S-cycling [6] . In our data, the abundance and activity of S-cycling groups—such as the Chromatiales , SAR324 and ARCTIC96BD-19 ( Fig. 3 and Fig. 6b )—are indicative of an active S-cycle in portions of the ETNP. At station 2 and 3, OMZ nitrite concentrations >1 μM (refs 22 , 27 ) fit the definition of an AMZ, and all of these groups were abundant. S cycling occurs off West Africa [5] , in the ETSP [6] , and may occur in the Arabian Sea [11] , and our data represent the first evidence of S cycling in the ETNP. Of particular note is the presence and activity of the Chromatiales : the most abundant Chromatiales OTU was 99% identical to 16S rRNA sequences previously collected in the ETNP (99% identical to accession numbers AY726856 and AY726933; ref. 13 ) and other major OMZs (99% identical to accession numbers EU092180 and DQ810641; refs 11 , 12 ). Collectively, these results suggest that Chromatiales are widely distributed in OMZs, and our data demonstrate that their abundances are tightly coupled to DO concentrations. Their role in OMZ S cycling deserves further attention. This represents one key group found in diverse communities present on the edge of the OMZ. Others found across the richest samples collected at each station in the ETNP include sixteen SAR11 OTUs, four SAR324 OTUs, two SAR406 OTUs, two Nitrospina OTUs and single NS2b marine Flavobacteria and ARCTIC96BD-19 OTUs. Within each of the high-richness samples, between 68 to 138 OTUs were not detected in any other sample. Sampling resolution may be a factor in the ETSP [10] and we acknowledge that this may influence our results as well: some of the OTUs detected within the high richness portions of the water column might be found in relatively thin, discrete layers not captured by our sampling. This highlights the need for highly-resolved sampling in OMZs, but MSDMs provide a computational approach to modelling the distribution of individual bacterial OTUs. Development of a cross-OMZ model would be valuable for examining differences among large open-ocean OMZs. In the ETNP, our MSDM results indicate that deoxygenation can alter the abundance patterns of hundreds of bacterial OTUs, with ~5% of OTUs responding to each 1 μmol kg −1 change in DO. Many of the groups that respond to simulated deoxygenation likely have important roles in C, N and S cycling within OMZs. We suggest that changes in their abundance, diversity and composition may have several downstream implications: First, organisms present in high-richness portions of the water column may act as regulators of fluxes of C, N and S into and out of the OMZ, and their rates of cycling and metabolism may respond to changing DO and light regimes. Our data indicate that their relative abundance is tightly coupled to environmental conditions and so will likely change with ocean warming and OMZ shoaling. Second, changing richness and evenness in microbial mesocosms can reduce aerobic respiration [17] and denitrification [20] rates, but whether this translates to functional changes in expanding OMZs is not yet known. Future research should quantify diversity–function relationships for key microbial biogeochemical processes in OMZs, and should they be identified, distinguish between ‘selection effects’ and complementarity [17] , [18] , [19] , [20] , [40] in driving such relationships. Third, N-cycling processes have well-documented sensitivity to DO and light that may be affected by OMZ shoaling. The high abundance of Nitrospina and high rates of nitrite oxidation within the OMZ may be affected by light [27] , potentially altering the form and availability of N for anaerobic processes in the OMZ (for example, decreasing the re-oxidation of nitrite back to nitrate). Fourth, S oxidation appears to be an important ecosystem service provided by microbes in OMZs [5] , and our data suggest that the composition of S-oxidizers changes with simulated deoxygenation. Whether this is indicative of functional redundancy and replacement has not been established, but will dictate the resiliency of this process to OMZ shoaling and deoxygenation. For all of these reasons, the aggregate effects of deoxygenation are complex, yet our gradient approach and use of MSDMs represent a first step to understanding these effects. Microorganisms are ultimately responsible for the decrease in DO with depth in the ocean [1] , [4] , biogeochemical models indicate that microbial responses are more important than physical factors in driving ocean deoxygenation [7] , and diverse bacterial communities found at the top of the OMZ likely have important roles in S oxidation [5] and coupled anaerobic and aerobic N cycling [4] , [9] . Changes in the functioning of these communities may have far-reaching effects on ocean biogeochemistry. Sample collection and oxygen measurements Samples were collected in July and August of 2008 aboard the R/V New Horizon in the GOC and eastern tropical North Pacific (ETNP). Six stations were occupied for several days each, and temperature, conductivity, chlorophyll and DO concentrations were measured using a Seabird SBE 9 CTD sensor package equipped with a Seapoint fluorometer and SBE oxygen sensor. Following initial test casts, samples were collected using 10 l bottles deployed on the CTD rosette; samples for DO and nutrient measurements were analysed within hours of collection to characterize the structure of the water column. Oxygen concentrations measured using the SBE oxygen sensor were corrected based on Winkler titrations ( r 2 =0.997, n =187 for the cruise). Depths of DNA/RNA sample collection were selected based primarily on oxygen and nutrient profiles: we sampled one to three depths straddling the base of the euphotic zone, followed by five to seven depths spaced every 5 m, and then four to six depths spaced every 10–20 m across the transition from hypoxic to suboxic conditions in the OMZ. Previous OMZ studies have used different sample collection approaches that may complicate direct comparisons, and may partly explain some differences among OMZs; Bryant et al . [10] , in particular, pre-filtered DNA samples and would not have captured particle-associated bacteria in their sampling. However, microbes in the free-living fraction are typically numerically dominant (>95% of total; ref. 41 ), such that peaks in richness likely reflect the diversity of free-living bacteria. DNA and RNA extraction At each depth, 4 l of seawater was collected from the CTD rosette and divided into two sets of 2 l samples, which were then filtered through separate 25 mm diameter 0.2 μm Suppor filters (Pall Corporation, Port Washington, NY, USA) using a peristaltic pump. Filters were flash frozen in liquid nitrogen and stored at −80 °C until DNA and RNA extraction, with one set of filters dedicated to each. Details of DNA extraction were reported in Beman et al . [22] Filters for RNA extraction were frozen in RLT buffer with beta-mercaptoethanol added (Qiagen, Valencia, CA, USA), and RNA was extracted using the Qiagen RNeasy kit, following Church et al . [42] , with the following modifications: tubes containing filters, glass beads and buffer were first agitated for 80 s on a FastPrep machine (MP Biomedicals, Solon, OH, USA) at setting 5.5; each sample and an equal volume of 70% ethanol solution was then bound to the RNeasy spin column, and purified and eluted following the manufacturer’s instructions. We used Turbo DNase (Ambion, Life Technologies Corporation, Carlsbad, CA, USA) to remove carry-over DNA; samples were treated with 10% DNase buffer and 5% DNase for 20 min at 37 °C. cDNA was generated from extracted RNA using the Invitrogen SuperScript III Reverse Transcriptase kit (Life Technologies Corporation, Carlsbad, CA, USA) following the manufacturer’s instructions. 10 μl of RNA extract, 1 μl each of random hexamers and 1 μl 10 mM dNTPs were incubated at 65 °C for 5 min, and then placed on ice for 1 min; samples were then incubated with 10 μl of cDNA synthesis mix (2 μl 10 × RT buffer, 4 μl 25 mM MgCl 2 , 2 μl 0.1M DTT, 1 μl RNase OUT (40 U μl −1 ) and 1 μl SuperScript III RT) for 25 °C for 10 min, then 55 °C for 50 min, and the RT reaction was terminated at 85 °C for 5 min. Remaining RNA was removed through incubation with RNase H (Invitrogen) at 37 °C for 20 min. Quantitative PCR Quantitative PCR (qPCR) assays were performed on a Stratagene MX3005P (Agilent Technologies, La Jolla, CA, USA) using the following reaction chemistry: 12.5 μl SYBR Premix F (Epicentre Biotechnologies, Madison, WI, USA), 2 mM MgCl 2 , 0.4 μM of each primer, 1.25 units AmpliTaq polymerase (Applied Biosystems, Life Technologies Corporation, Carlsbad, CA, USA), 40 ng μl −1 BSA, and 1 ng DNA in a final volume of 25 μl. 16S rRNA genes from Nitrospina were amplified using the primers NitSSU_130F (5′-GGGTGAGTAACACGTGAATAA-3′) and NitSSU_282R (5′-TCAGGCCGGCTAAMCA-3′) (ref. 43 ). Cycling conditions were modified from Mincer and et al . [43] : the total number of cycles was reduced from 50 to 30, and the length of the detection step was increased from 1 to 7 s. The partial 16S rRNA sequence from the uncultured marine Nitrospinaceae bacterium recovered on BAC EB080L20_F04 (ref. 43 ) was used as a QPCR standard; this sequence was synthesized at Blue Heron Biotechnologies (Bothell, WA, USA) and used in tenfold dilutions from 10 7 to 10 2 16S rRNA genes per μl to generate standard curves ( r 2 =0.987–0.994). Chromatiales 16S rRNA PCR was conducted on cDNA generated from RNA samples collected in the OMZ at stations 2–5. The Chromatiales -specific primer Chr986f (5′-AGCCCTTGACATCCTCGGAA-3′) from Coolen and Overmann [44] and universal bacterial primer 1392R (5′-ACGGGCGGTGTGTAC-3′) were used to amplify Chromatiales 16S rRNA. We used cycling conditions from Coolen and Overmann [44] (95 °C for 4 min; followed by 15 cycles of 94 °C for 30 s, 65 °C for 90 s, and 72 °C for 40 s; and 25 cycles of 94 °C for 30 s, 58 °C for 60 s, and 72 °C for 40 s) and did not directly quantify 16S rRNA genes, but instead monitored amplification during real-time PCR. DNA from 14 m depth in Jellyfish Lake in the Republic of Palau was used as a positive control: this anoxic lake has a well-defined plate of purple sulphur bacteria that is visually observable [45] and that was sampled in August 2010. Pyrosequencing indicated a large proportion of 16S rRNA genes in this sample belonged to the Chromatiales (Beman, Meyerhof and Dawson, manuscript in preparation). For all QPCR assays, product specificity was verified via dissociation curves, and multiple negative controls (nuclease-free water) were included in each run, none of which exhibited amplification. Pyrosequencing approach DNA samples were sequenced using Titanium chemistry on the Roche 454 FLX platform at Research and Testing Laboratories (Lubbock, TX, USA). Bacteria-specific primer 27F (5′-GAGTTTGATCNTGGCTCAG-3′) and universal primer 519 R (5′-GWNTTACNGCGGCKGCTG-3′) [46] were modified with additional degeneracies (Ns in primer sequence) and used to amplify a portion of the bacterial 16S rRNA gene. Based on ARB SILVA TestPrime ( http://www.arb-silva.de/search/testprime/ ; [47] ), these primers amplify 88.9% of eligible bacterial 16S rRNA sequences in the ARB SILVA database, with no bias among dominant bacterioplankton phyla such as the Proteobacteria , Cyanobacteria , Actinobacteria and Bacteroidetes . Relevant linkers were attached to primers, as were 8-base barcodes [48] used to sort individual samples. We used the program mothur ( http://www.mothur.org [49] ;) for all sequence analyses, and for the 60 samples, we recovered 714,245 sequences with a median read length of 475 bp. Following the approach of Huse et al . [50] for quality control, we discarded sequences: >±100 bp from the median sequence length, containing any ambiguous bases, containing homopolymers >8 bp, of <25 average quality score, and that did not exactly match the forward primer and barcode sequence. Of the sequences that were removed, the majority were removed because they did not exactly match the forward primer and barcode. (We did not screen sequences based on the reverse primer, as some of the reads are high-quality sequences that did not extend to the reverse primer.) In total, 282,030 sequences did not meet quality control criteria and were excluded from subsequent analyses. Bacterial 16S rRNA sequences were aligned to the greengenes alignment [51] in mothur. The alignment was optimized to the start position and we discarded sequences starting after the position that 95% of the sequences start; the alignment was then manually curated to remove misaligned sequences ( n =25). Kunin et al . [52] raised the issue of pyrosequencing errors inflating diversity estimates, and Huse et al . [53] proposed a pseudo-single linkage ‘preclustering’ algorithm as a means of reducing these errors; we used this approach as implemented in mothur to remove OTUs that may be produced by pyrosequencing errors. In addition, we analysed much longer sequences (475 bp versus 60–110 bp for ‘pyrotags’), and calculated diversity indices at 97% identity, to avoid error-inflated diversity estimates. A total of 408,013 16S rRNA sequences were subsequently analysed, and individual sample library size ranged from 1,298 sequences to 12,811 sequences, with an average of 6,800 (±2,563 s.d.). Libraries from 100 and 150 m depth at station 6 contained 1,298 and 2,061 sequences, respectively, and were the only libraries containing <3,000 sequences. As the two smallest libraries were present at the same station, we elected to normalize all libraries to 1,298 sequences despite the loss of sequence information. Overall trends for libraries normalized to 3,000 sequences are highly consistent with those normalized to 1,298 (for example, compare Table 1 and Supplementary Table S1 ): correlation coefficients were similar, and measured and estimated richness declined at <20 μmol kg −1 DO ( Supplementary Table S1 , Supplementary Fig. S5 ). Libraries were normalized by randomly removing sequences to reduce the total number of sequences in each library to a common size. Diversity indices (observed richness, ACE, Shannon, Gini) were calculated for libraries at 97% sequence identity using average neighbour clustering. Beta diversity calculations were performed across these samples and changes in community composition were explored using the abundance-based Sørensen index. Taxonomic composition of individual samples was determined by classification of 16S rRNA sequences based on the ARB SILVA data set [54] in mothur, and data are reported for a consensus confidence threshold of 65%. Deoxygenation rates Previous work has used historical oxygen measurements differenced from recent observations to calculate deoxygenation rates in the Eastern tropical Atlantic [3] ; we used the same approach but calculated a single rate based on differences between our cruise data and historical data from the CalCOFI database. Based on queries of the World Ocean Database ( http://www.nodc.noaa.gov/OC5/SELECT/dbsearch/dbsearch.html ), which is the basis for the World Ocean Atlas, CalCOFI data collected in 1956–1957 represent the earliest oceanographic data collected in the GOC/ETNP. We extracted these data from the CalCOFI database ( http://www.calcofi.org/ ), and calculated deoxygenation rates based on differences in oxygen concentrations between 2008 cruise data and 1956–1957 CalCOFI data, following Stramma et al . [8] : we assumed a linear decrease, and integrated over the 300–700 m depth interval assuming a nominal density of 1027.2 kg m −3 . Uncertainty in our oxygen data is derived from the CTD’s SBE oxygen sensor (2% accuracy) and the Winkler titrations used to correct CTD data, which have an uncertainty of 2.1% based on repeated measurements of calibrations. We assume that CalCOFI measurements have similar uncertainty. MARS and SDMs SDMs have gained wide applicability and acceptance in ecology [29] , [30] and are now being adapted to microbial communities [18] . MARS [28] is ideal for microbial SDMs, because it is not constrained to presence-only data sets, can be used quantitatively (rather than just modelling presence-absence, as is common for other SDM approaches [30] ) and can incorporate species interactions within the community [31] . We modelled OTU abundances based on DO concentrations at set depth intervals (those used by WOA and CalCOFI) and all data collected by the CTD (including DO), and evaluated the model based on correlations between observed and modelled OTU abundances. For the DO-only model, we found strong correlation between observed and modelled OTU abundances for the 77 most abundant OTUs (average r 2 =0.54, range of 0.28–0.81). For purposes of comparison with macrobial SDMs, these values correspond to area under the receiver operating characteristic curve (AUC) values of 0.41–1, with a mean of 0.85. The SDM yielded perfect AUC values for OTUs 8 (a SAR11 OTU), 14 (SAR11), 25 ( Acidobacteria ), 28 ( Nitrospina ), 37 ( Rhodobacteria ) and 71 (SAR324). r 2 values were more variable for OTUs 78-2602, ranging from 0 to 0.85, with an overall mean of 0.23. All OTUs beyond 2602 were singletons observed only once in the sequencing data set; as would be expected, the SDM provided mixed results depending on the depth/samples where the singletons were detected. Highest r 2 values (>0.3) were observed for many of the richest samples (400 and 700 m at station 1, 150 m at station 2, 140 m at station 4 and 100–200 m at station 5), which most likely reflects how MARS basis functions were constructed based on DO, and the fact that, across stations, half of our samples spanned the DO gradient of 1 to 40 μmol kg −1 . Many singleton OTUs had AUC scores of 1—that is, the SDM accurately modelled the depth where they were detected—but the SDM sometimes overpredicted the presence of singletons. This suggests that our results are likely conservative in terms of changing richness. The SDM based on all CTD data was more robust, with r 2 values of 0.16–0.99, with a mean of 0.59 across all non-singleton OTUs. For individual samples, r 2 values for the comparisons between observed and modelled OTU abundances ranged from 0.82–0.99, with a mean r 2 of 0.96. Put another way, for each sample over 82% of the variability in relative abundance of different OTUs was captured by the SDM. This performance reflects the larger number of input variables as well as the fact that MARS can capture biological interactions [31] . As some of these variables were not collected historically (for example, PAR and transmission) this model could not be applied to past data. Oceanographic data were visualized in Ocean Data View ( http://odv.awi.de/ ) and statistical analyses were conducted in MINE, MATLAB and in R (using the mda and vegan packages). Accession Codes: DNA sequence data derived here have been deposited in the Sequence Read Archive ( SAMN01942182 ). How to cite this article: Beman, J. M. et al . Deoxygenation alters bacterial diversity and community composition in the ocean’s largest oxygen minimum zone. Nat. Commun. 4:2705 doi: 10.1038/ncomms3705 (2013).